Bond cleavage, fragment modification and reassembly in enantioselective three-component reactions Chemical bond cleavage and reconstruction are common processes in traditional rearrangement reactions. In contrast, the process that involves bond cleavage, fragment modification and then reconstruction of the modified fragment provides an efficient way to build structurally diversified molecules. Here, we report a palladium(II)/chiral phosphoric acid catalysed three-component reaction of aryldiazoacetates, enamines and imines to afford α-amino-δ-oxo pentanoic acid derivatives in good yields with excellent diastereoselectivities and high enantioselectivities. The stereoselective reaction went through a unique process that involves cleavage of a C–N bond, modification of the resulting amino fragment and selective reassembly of the modified fragment. This innovative multi-component process represents a highly efficient way to build structurally diversified polyfunctional molecules in an atom and step economic fashion. A keto-iminium is proposed as a key intermediate and a chiral palladium/phosphate complex is proposed as an active catalyst. Innovative processes involving new modes of chemical bond formation are highly desirable to achieve challenging synthetic tasks that existing ones cannot easily accomplish [1] . Rearrangement reactions, for example, have been intensively investigated to provide a unique way to build one molecule from its mother molecule in a 100% atom-efficient fashion [2] . Bond cleavage and reconstruction involved in the rearrangement reactions occur in the same molecule [3] , [4] , [5] and typically in a concerted fashion ( Fig. 1 path a) [2] . In addition, bond cleavage and reassembly of fragments in traditional two-component reactions have been reported [6] , [7] , [8] , [9] , [10] , but in most cases, these reactions resulted in either loss of components [8] or random combination of the fragments such as radical fragments without any selectivity [9] , [10] . We communicate here a multi-component process that involves chemical bond cleavage, fragment modification and specific reassembly of the modified fragment to afford functional group-enriched molecules ( Fig. 1 path b). This innovative process provides a unique way to build diversified molecules in an efficient and atom-economic fashion. 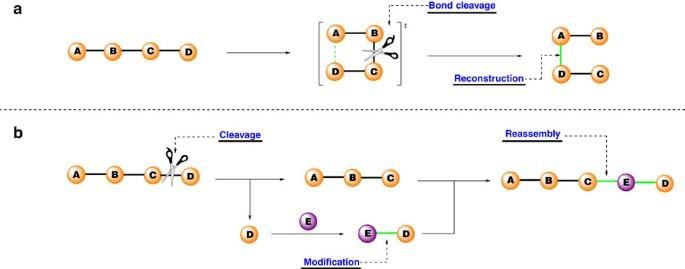Figure 1: Conceptual framework. (a) Intramolecular rearrangement: bond cleavage and reconstruction. (b) Concept of bond cleavage, fragment modification and reassembly. Figure 1: Conceptual framework. ( a ) Intramolecular rearrangement: bond cleavage and reconstruction. ( b ) Concept of bond cleavage, fragment modification and reassembly. Full size image We have recently reported an efficient trapping process in which zwitterionic intermediates were trapped by electrophiles to produce polyfunctional molecules in a single synthetic step [11] , [12] . In the reported reactions, for example, indoles and pyrroles containing a cyclic enamine as a key structural motif were successfully employed as substrates ( Fig. 2a ). In continuation with this study, we envisioned that using an acyclic enamine should undergo a similar transformation to afford a zwitterionic intermediate trapping product ( Fig. 2b ) [13] . Thus, the three-component reaction of methyl phenyldiazoacetate, an acyclic enamine and an imine was conducted. However, the proposed process did not occur as expected, but we discovered a novel process that involves cleavage of a C–N bond, modification of the resulting amino fragment by forming an ammonium ylide and regio- and stereoselective reassembly of the modified fragment back to another iminium fragment to produce a chiral α-amino-δ-oxo pentanoic acid derivative ( Fig. 2c ). In this three-component reaction, one bond cleavage and three bonds formation take place in one step to produce a new molecule bearing two stereogenic centres including one quaternary carbon centre in excellent diastereoselectivity and high enantioselectivity. This unique process provides an easy access for highly efficient construction of chiral α-amino-δ-oxo pentanoic acid derivatives [14] , [15] , [16] , [17] from simple substrates under mild reaction conditions. 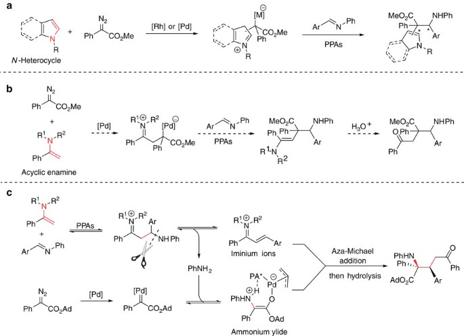Figure 2: Discovery of the novel process. (a) Prior works for the enantioselective trapping of zwitterionic intermediates. (b) Hypothetical pathway for the enamine-participated multi-component reaction. (c) Actual process: bond cleavage, fragment modification and reassembly. Figure 2: Discovery of the novel process. ( a ) Prior works for the enantioselective trapping of zwitterionic intermediates. ( b ) Hypothetical pathway for the enamine-participated multi-component reaction. ( c ) Actual process: bond cleavage, fragment modification and reassembly. Full size image Preliminary optimization Initial reaction of methyl phenyldiazoacetate 2a , enamine 3a and imine 4a was carried out in dichloromethane (CH 2 Cl 2 ) at ambient temperature under the catalysis of [PdCl( η 3 -C 3 H 5 )] 2 and Brønsted acid rac - 1a . After hydrolysis, product 5a was obtained in just 15% isolated yield with excellent diastereoselectivity (>95:5 diastereomeric ratio, dr) accompanying with 35% of side product 1,5-diketo 6 ( Table 1 , entry 1). The structural identity of 5a was later confirmed by single-crystal X-ray analysis (see Supplementary Fig. 63 ). The interesting process for the formation of 5a attracted us for further studies. To suppress the formation of the side product 6 , minimizing the concentration of 3a in the reaction mixture was thought to be critical. Thus, a solution of 2a and 3a was slowly introduced to the reaction mixture over 1 h. As a result, the yield of 5a was increased to 45% ( Table 1 , entry 2). The product yield of 5a was further enhanced to 63% and side product 6 was decreased to 6% yield by performing the reaction in an ice-bath ( Table 1 , entry 3). Lowering the reaction temperature to −20 °C resulted in a very slow process for the diazo decomposition and no improved results were obtained ( Table 1 , entry 4). Table 1 Preliminary results for the title three-component reaction*. Full size table Enantioselective reaction We then explored the enantioselective control of the novel process. A series of chiral 3,3’-disubstituted BINOL-derived phosphoric acids (PPAs) [11] , [12] were tested and the results were summarized in Table 2 . Bulky substituted phosphoric acids 1b and 1c were found to be less effective to promote this reaction, as only trace amount of product was observed ( Table 2 , entries 1–2). Moderate-to-good enantioselectivities were obtained by using PPAs 1d – 1k (upto 80:20 enantiomeric ratio (er), entries 3–10, Table 2 ). Other solvents did not improve the er further in this case (see Supplementary Table 1 ). To further improve the enantioselectivity, a more sterically hindered diazo compound tert -butyl phenyldiazoacetate 2b was used. While a sharp drop in enantiomeric excess (ee) value was observed with PPA 1e , less bulkier PPA 1i gave the product with increased er to 82:18 ( Table 2 , entry 11 versus 12). Additional reaction condition optimization increased the er to 92:8 when chloroform (CHCl 3 ) was used as the solvent at a reaction temperature of −20 °C ( Table 2 , entry 14). When the extremely bulky diazo compound 2c was used, the reaction proceeded in CHCl 3 at −10 °C to give 5a in 69% yield, >95:5 dr and 94:6 er ( Table 2 , entry 16). Table 2 Optimization for the enantioselective three-component reaction of 2 and 3a with 4a*. Full size table Substrate scope With optimized reaction conditions identified, the substrate scope of the reaction was explored. 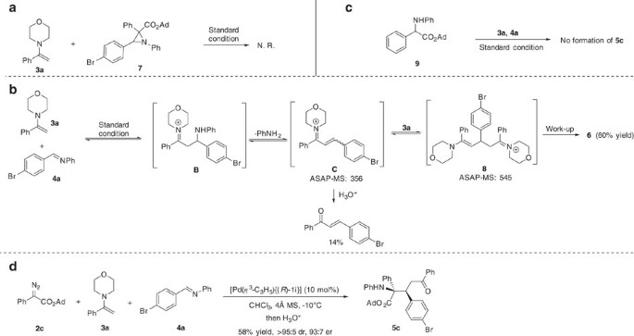Figure 3: Discussion on the reaction pathway. (a) Control reaction to exclude the formation of5cfrom aziridine7. (b) Proposed reaction pathway for the formation of6via iminium intermediateC. (c) Control reaction to exclude the formation of5cfrom N–H insertion product9. (d) Reaction under the catalysis of a premade palladium/phosphate complex to confirm the active catalyst. With respect to the imine substrate, the reactions gave good yields with high-to-excellent dr and er ( Table 3 , entries 1–10). The best result came from electron-deficient imine 4b , which gave product 5d in 65% yield with 95:5 dr and 96:4 er ( Table 3 , entry 2). The reaction was extended to other aryldiazoacetates ( Table 3 , entries 11–15) and enamines ( Table 3 , entries 16–17). All the reactions gave comparably good results except for diazo compound 2f , which bears three electron-donating methoxyl groups, resulting in product 5o with decreased er to 73:27 ( Table 3 , entry 13). For a representative example, with 4-fluoro substituted enamine 3c , the reaction gave corresponding product 5s in 64% isolated yield with 96:4 dr and 97:3 er ( Table 3 , entry 17). Table 3 Substrate scope of enantioselective three-component reaction of 2 and 3 with 4*. Full size table To understand the reaction pathway for this new process, several control experiments were initially performed. Aziridination product 7 was first isolated from the reaction of diazo compound 2c and imine 4a . Then treatment of aziridine 7 with enamine 3a did not give any ring opening product ( Fig. 3a ). This experiment excluded the possibility that the product 5c was resulted from a stepwise reaction pathway via intermediate 7 . In addition, in the absence of the diazo compound, the reaction gave side product 6 in a 60% yield together with a 14% yield of chalcone (chalcone is inactive in trapping of ammonium ylide under current conditions, see Supplementary Figure 65 ). Process of the above Mannich-type reaction from the addition of 3a to 4a was monitored by 1 H NMR, and it was found that concentration of liberated free aniline increased along with the reaction proceeding, which indicates that a retro aza-Michael addition to cleave the C–N bond does occur (see Supplementary Fig. 67 ). The cleavage of the C–N bond is also consistent with the formation of side product 6 as proposed in the following reaction pathway ( Fig. 3b ): (1) a Mannich-type addition of enamine 3a to imine 4a gives its adduct B ; (2) a C–N cleavage occurs through a retro aza-Michael addition to give a keto-iminium intermediate [18] , [19] , [20] , [21] C and an aniline fragment; (3) a conjugated addition of another enamine 3a to the keto-iminium produces the intermediate 8 ; (4) hydrolysis work-up of 8 produces the side product 6 . In addition, the keto-iminium intermediate was detected by Atmospheric Solids Analysis Probe Mass Spectrometry (ASAP-MS) (see Supplementary Fig. 66 ). All the information shown above indicates that the C–N bond cleavage does not need any assistance of a metal carbene. To rule out the possibility that product 5c was resulted from stepwise reactions of an N–H insertion of the free aniline and then a Michael-type addition to iminium intermediate C, an additional control experiment by addition of the premade N–H insertion product 9 to the reaction mixture was conducted, and no 5c was observed ( Fig. 3c ). The concerted reaction pathway is in agreement with our previous studies in the trapping of active ylides by other electrophiles [22] . Finally, to get information regarding active catalytic species, the crude reaction mixture was subjected to the high-resolution mass spectrum (HRMS). The palladium/phosphate complex [Pd(allyl)( 1i )] ([M+1] + : 918.8259, see Supplementary Fig. 72 ) was detected in the HRMS analysis. To further confirm the critical role of the chiral palladium/phosphate complex, [Pd(allyl)( 1i )] ( Supplementary Figure 73 and Supplementary method 3 ) was prepared [12] and used in the reaction of 2c , 3a and 4a . Product 5c was obtained in 58% yield with exactly the same stereoselective control of 95:5 dr and 93:7 er ( Fig. 3d versus entry 6 in Table 3 ), indicating that the palladium/phosphate complex is the real catalyst in the catalytic cycles. Figure 3: Discussion on the reaction pathway. ( a ) Control reaction to exclude the formation of 5c from aziridine 7 . ( b ) Proposed reaction pathway for the formation of 6 via iminium intermediate C . ( c ) Control reaction to exclude the formation of 5c from N–H insertion product 9 . ( d ) Reaction under the catalysis of a premade palladium/phosphate complex to confirm the active catalyst. Full size image On the basis of the information above, a plausible mechanism is proposed in Fig. 4 . First, reaction of an imine, a phosphoric acid and allylpalladium(II) chloride dimer gives iminium A and generates palladium/phosphate complex [Pd(allyl)PA*] as an active catalyst. Nucleophilic addition of an enamine 3 to the iminium A affords a Mannich-type adduct B as a ‘mother’ molecule. We propose that a retro aza-Micheal addition occurs here to cleave the C–N bond and produce an aniline fragment Ar 3 NH 2 and conjugated iminium intermediate C as a ‘mother’ fragment (cycle I). In the meantime, in the catalytic cycle II, [Pd(allyl)PA*] catalyzes diazo decomposition of 2 generating a palladium carbenoid D by the extrusion of dinitrogen. Modification of the aniline fragment by reacting with the carbenoid D gives a proposed Pd-associated ammonium ylide E or its enolate form F . Then, reassembly of the ammonium ylide back to the ‘mother’ fragment C via an enantioselective Michael-type addition produces an enamine intermediate G and regenerates [Pd(allyl)PA*] catalyst. Finally, hydrolysis of G during work-up affords the final products 5 . 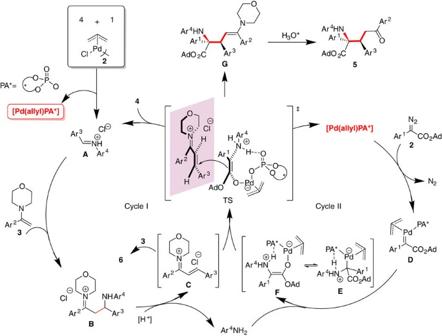Figure 4: Putative reaction pathways. Cycle I: formation of iminium salt C; cycle II: formation of ammonium ylides. Figure 4: Putative reaction pathways. Cycle I: formation of iminium salt C; cycle II: formation of ammonium ylides. Full size image To further confirm the C–N bond cleavage of the mother molecule B producing iminium intermediates C and eliminating the aniline fragment, p -bromoaniline was introduced to the reaction and the control experiment gave the cross-coupling product 10 in 17% yield ( Fig. 5a ), supporting the existence of fragments C (for other cross-coupling reactions, see Supplementary Figs 68–70 ). The existence of enamine intermediate G can be confirmed by direct detection by ASAP-MS ([M+H] + : 717, see Supplementary Fig. 71 ) and by reduction of the crude reaction mixture to corresponding amine derivatives. Treatment of the crude product mixture with NaBH(OAc) 3 /AcOH afforded α,δ-diamino acid derivatives 11a and 11b in 59% yield with 55:45 dr ( Fig. 5b ). The absolute configuration of 11b was confirmed as (2 R , 3 S, 5 R ) by X-ray single-crystal analysis (see Supplementary Fig. 64 ) and that of 5 was determined as (2 R , 3 S ) by analogy. 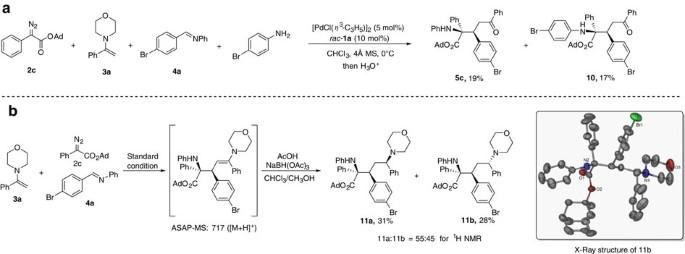Figure 5: The additional evidence and structure determination. (a) Cross-coupling control experiment reaction to confirm the C–N bond cleavage. (b) Reduction of enamine intermediateGto diamines11aand11b, and the structure determination of11bby single-crystal X-ray diffraction analysis. Figure 5: The additional evidence and structure determination. ( a ) Cross-coupling control experiment reaction to confirm the C–N bond cleavage. ( b ) Reduction of enamine intermediate G to diamines 11a and 11b , and the structure determination of 11b by single-crystal X-ray diffraction analysis. Full size image Since the retro aza-Michael addition is considered to be a reversible process, it is still possible that the product formation is directly through the Mannich product B via a ylide formation from B and followed by a 1,2-C shift. To evaluate this possibility, density functional theory calculation was carried out. A reaction pathway involving the ylide formation and the 1,2-C shift is exothermic by 24.3 kcal mol −1 . However, this pathway has to proceed through a transition state with a higher energy than that of the B by 21.9 kcal mol −1 and surmounts an energy barrier of 29.4 kcal mol −1 , which is considered to be unfavourable in thermodynamics (see Supplementary Figs 74–77 ). In conclusion, we report an enantioselective three-component reaction of diazo compounds, enamines and imines. This reaction proceeds through an innovative process that involves C–N cleavage, modification of the amino fragment and selective reassembly of the modified fragment. This unique process provides a convenient pathway to chiral α-amino-δ-oxo pentanoic acid derivatives in good yields and high stereoselectivities. Mechanistic study reveals that a keto-iminium fragment is the key intermediate and a chiral palladium/phosphate complex is the real catalyst. This innovative mode of bond formation provides an atom-efficient and step-economic way to build functional group-enriched molecules that existing methods cannot easily accomplish, and could inspire more discoveries in the efficient construction of unique molecules. General 1 H NMR (400 MHz), 13 C NMR (100 MHz) and 19 F NMR (376 MHz) spectra were recorded on Brucker Asend 400 spectrometers. HRMS was performed on Waters Micromass Q-TOF micro Synapt High Definition Mass Spectrometer. HPLC analysis using a chiral stationary phase was performed on Shimadzu or Dalian Elite (UV230+ UV/Vis Detector and P230P High Pressure Pump). CHIRALCEL OD-H or CHIRALPAK IC column was purchased from Daicel Chemical Industries, Ltd. Single-crystal X-ray diffraction data were recorded on Bruker-AXS SMART APEX II single-crystal X-ray diffractometer. See Supplementary Figs 1–62 for the NMR spectra and HPLC chromatograms, Supplementary Table 1 for the optimization of reaction, Supplementary Discussion for the mechanism studies and computational details and Supplementary Methods for the characterization data of compounds not listed in this part. Materials THF and toluene were distilled over sodium. CH 2 Cl 2 and CHCl 3 were distilled over calcium hydride. Enamines 3 were synthesized from acetophenone and morpholine [13] . Diazo compounds were prepared according to the literature [12] , [23] . Aldimines 4 were prepared from condensation of the corresponding aldehydes with arylamines according to the reported methods [24] . Chiral BINOL-derived phosphoric acids ( 1a – 1k) were prepared according to the literature procedures [11] , [12] . General procedure for enantioselective three-component reactions A suspension of [PdCl( η 3 -C 3 H 5 )] 2 (3.6 mg, 5.0 mol%), chiral phosphoric acid ( R )- 1i (15 mg, 10 mol%), imine 4 (0.2 mmol, 1.0 equivalent (eq)) and 4 Å molecular sieve (0.2–0.3 g) was stirred in 1.5 ml of CHCl 3 in a test tube equipped with plug at −10 °C. The mixture of diazo compound 2 (0.3 mmol, 1.5 eq) and enamine 3 (0.22 mmol, 1.1 eq) in 1.0 ml CHCl 3 was introduced to the suspension over 1 h via a syringe pump. After completion of the addition, the mixture was stirred for another 5 min and then was hydrolyzed by elution through short column chromatography on silica gel (eluent: EtOAc/petroleum ether=1/10~1/5) to give a crude product, which was subjected to 1 H NMR spectroscopy analysis for the determination of diastereoselectivity and to chiral HPLC analysis for the ee values. Purification of the crude products by flash chromatography on silica gel (eluent: EtOAc/petroleum ether=1/80~1/20) afforded pure products. (2 R ,3 S )-adamantan-1-yl 3-(4-bromophenyl)-5-oxo-2,5-diphenyl-2-(phenylamino)pentanoate (5c) Obtained following the general procedure in 69% yield (89 mg). 1 H NMR (400 MHz, CDCl 3 ) δ 7.75–7.66 (m, 2H), 7.64–7.56 (m, 2H), 7.48 (dd, J =10.5, 4.3 Hz, 1H), 7.39–7.29 (m, 7H), 7.09–7.02 ( m, 1H), 6.68 (m, 1H), 6.41 (d, J =7.8 Hz, 1H), 4.88 (s, 1H), 4.62 (dd, J =11.4, 2.2 Hz, 1H), 3.61 (dd, J =17.4, 11.5 Hz, 1H), 3.41 (dd, J =17.4, 2.4 Hz, 1H), 2.04 (s, 3H), 1.76 (q, J =11.4 Hz, 6H), 1.62–1.41 (m, 6H); 13 C NMR (100 MHz, CDCl 3 ) δ 197.5, 171.0, 145.7, 137.8, 137.3, 136.7, 133.2, 131.6, 131.0, 128.6, 128.5, 128.3, 127.9, 127.7, 121.4, 117.8, 115.9, 82.8, 70.1, 48.3, 40.9, 40.8, 36.0, 30.7; FT-IR (KBr) 3,404; 3,052; 2,912; 2,852; 1,728; 1,687; 1,600; 1,502; 1,447; 1,354; 1,322; 1,259; 1,235; 1,176; 1,073; 1,053; 965, 747, 696, 684 cm −1 . HRMS(ESI) m/z : calculated (calcd.) for C 39 H 38 NO 3 NaBr (M+Na) + 670.1933, found 670.1929. HPLC (CHIRALCEL OD-H, λ = 254 nm, hexane/2-propanol=99/1, flow rate=1.0 ml min −1 ), 88–90% ee, t major =5.74 min, t minor =8.47 min. Procedure for the preparation of 11a and 11b A suspension of [PdCl( η 3 -C 3 H 5 )] 2 (7.2 mg, 5.0 mol%), chiral phosphoric acid ( R )- 1i (30 mg, 10 mol%), imine 4a (105 mg, 0.4 mmol, 1.0 eq) and 4 Å molecular sieve (0.1 g) was stirred in 2 ml of CHCl 3 at −10 °C, and then the mixture of diazo compound 2c (199 mg, 0.6 mmol, 1.5 eq) and enamine 3a (84 mg, 0.44 mmol, 1.1 eq) in 1.5 ml CHCl 3 was introduced to the suspension over 1 h via a syringe pump. After completion of the addition, the mixture was stirred for another 10 min. To the mixture, NaBH(OAc) 3 (5.0 eq. ), AcOH (0.4 ml) and CH 3 OH (3 ml) were added at −10 °C and stirred at room temperature. After the reaction completed (monitored by TLC), the mixture was filtered through Celite. The filtrate was concentrated down to give a residue, which was subjected to 1 H NMR for determination of dr and was purified by flash chromatography on silica gel (eluent: EtOAc/petroleum ether=1/80~1/10) to afford pure 11a and 11b . (2 R ,3 S ,5 R )-adamantan-1-yl 3-(4-bromophenyl)-5-morpholino-2,5-diphenyl-2-(phenylamino)pentanoate (11a) A total 32% yield (92 mg); [ α ] =−43.0 ( c =0.348, CHCl 3 ); 1 H NMR (400 MHz, CDCl 3 ) δ 7.67 (d, J =3.9 Hz, 2H), 7.35 (d, J =8.3 Hz, 2H), 7.32–7.26 (m, 3H), 7.22 (dt, J =10.7, 4.0 Hz, 3H), 7.03–6.95 (m, 2H), 6.92–6.78 (m, 4H), 6.68–6.57 (m, 1H), 6.37 (d, J =8.0 Hz, 2H), 4.61 (s, 1H), 4.16 (d, J =11.0 Hz, 1H), 3.67 (t, J =4.4 Hz, 4H), 2.87 (dd, J =11.7, 3.1 Hz, 1H), 2.54 (t, J =12.0 Hz, 1H), 2.35–2.20 (m, 2H), 2.03 (s, 3H), 1.98–1.89 (m, 2H), 1.83 (dd, J =19.0, 7.1 Hz, 1H), 1.76–1.65 (m, 6H), 1.58–1.38 (m, 7H); 13 C NMR (100 MHz, CDCl 3 ) δ 171.5, 145.9, 138.1, 137.5, 137.2, 131.9, 131.0, 129.6, 128.5, 128.4, 127.9, 127.5, 127.4, 121.2, 117.9, 115.7, 82.2, 77.3, 77.0, 76.7, 70.7, 67.6, 65.9, 52.1, 49.2, 40.8, 36.0, 32.0, 30.7. FT-IR (KBr) 3,416; 3,056; 3,026; 1,725; 1,703; 1,604; 1,501; 1,452; 1,355; 1,317; 1,254; 1,230; 1,182; 1,118; 1,051; 1,108; 967, 822, 751, 703, 553 cm −1 ; HRMS(ESI) m/z : calcd. for C 43 H 48 N 2 O 3 Br (M+H) + 719.2848, found 719.2876. (2 R ,3 S ,5 S )-adamantan-1-yl 3-(4-bromophenyl)-5-morpholino-2,5-diphenyl-2-(phenylamino)pentanoate (11b) A total 28% yield (80 mg); 1 H NMR (400 MHz, CDCl 3 ) δ 7.41–7.31 (m, 6H), 7.31–7.19 (m, 4H), 7.03–6.91 (m, 4H), 6.74–6.53 (m, 3H), 6.28 (d, J =7.8 Hz, 2H), 4.44 (s, 1H), 3.61–3.44 (m, 1H), 3.14 (d, J =10.5 Hz, 1H), 2.58 (dd, J =11.2, 3.2 Hz, 1H), 2.41 (td, J =12.9, 3.3 Hz, 1H), 2.26–2.12 (m, 3H), 2.11–2.02 (m, 2H), 1.99 (s, 3H), 1.66–1.56 (m, 6H), 1.56–1.43 (m, 6H); 13 C NMR (100 MHz, CDCl 3 ) δ 171.0, 145.7, 139.4, 137.1, 136.5, 131.9, 131.0, 129.6, 129.1, 128.4, 128.3, 127.67, 127.5, 127.4, 121.5, 117.8, 115.7, 82.2, 77.3, 77.0, 76.7, 70.5, 68.6, 67.0, 51.4, 40.6, 36.0, 33.6, 30.7; FT-IR (KBr) 3,390; 3,059; 3,026; 2,955; 2,911; 2,852; 2,812; 1,713; 1,604; 1,500; 1,450; 1,258; 1,233; 1,181; 1,119; 1,054; 1,010; 876, 821, 759, 703, 547 cm −1 ; HRMS(ESI) m / z : calcd. for C 43 H 48 N 2 O 3 Br (M+H) + 719.2848, found 719.2833. How to cite this article : Zhang, D. et al. Bond cleavage, fragment modification and reassembly in enantioselective three-component reactions. Nat. Commun. 6:5801 doi: 10.1038/ncomms6801 (2015). Accession codes: The X-ray crystal structure information is available at the Cambridge Crystallographic Data Centre (CCDC) under deposition numbers CCDC-981292 (5a) and CCDC-999727(11b). These data can be obtained free of charge from The Cambridge Crystallographic Data Centre via www.ccdc.cam.ac.uk/data_request/cif